Measurement and control of quasiparticle dynamics in a superconducting qubit Superconducting circuits have attracted growing interest in recent years as a promising candidate for fault-tolerant quantum information processing. Extensive efforts have always been taken to completely shield these circuits from external magnetic fields to protect the integrity of the superconductivity. Here we show vortices can improve the performance of superconducting qubits by reducing the lifetimes of detrimental single-electron-like excitations known as quasiparticles. Using a contactless injection technique with unprecedented dynamic range, we quantitatively distinguish between recombination and trapping mechanisms in controlling the dynamics of residual quasiparticle, and show quantized changes in quasiparticle trapping rate because of individual vortices. These results highlight the prominent role of quasiparticle trapping in future development of superconducting qubits, and provide a powerful characterization tool along the way. Superconducting quantum circuits have made rapid progress [1] in realizing increasingly sophisticated quantum states [2] , [3] and operations [4] , [5] with high fidelity. Excitations of the superconductor, or quasiparticles (QPs), can limit their performance by causing relaxation and decoherence, with the rate approximately proportional to the QP density [6] . Operating at 20 mK or lower temperature, superconducting aluminium in thermal equilibrium should have no more than one QP for the volume of the Earth. However, a substantial background of QPs has been observed in various devices from single electron [7] or Cooper-pair transistors [8] , kinetic inductance detectors [9] , [10] to superconducting qubits [11] , [12] , [13] . A detailed understanding of the generation mechanism and dominant relaxation processes will eventually be necessary to suppress this small background of QPs and continue the improvement of these devices. QP dynamics has been traditionally characterized by the ‘lifetime’ of excess QPs relaxing towards a steady state, τ ss . A variety of techniques have been used to measure τ ss in aluminium, including low-frequency sub-gap electrical [14] , [15] or thermal transport [16] , [17] , resonance frequency shifts [18] , [19] and more recently, qubit energy decay [20] , [21] . Electron–phonon-mediated pair recombination has been established as the canonical mechanism of QP decay [22] . Single-QP loss mechanisms in the presence of QP ‘traps’, such as normal metal contacts [7] , [16] , [17] , [23] , [24] , engineered gap inhomogeneity [8] , [25] , [26] , Andreev bound states [27] or magnetic field penetration [28] , [29] , have also been studied. Ascertaining the relative importance of QPs to the decoherence of any superconducting qubit, versus other mechanisms such as dielectric loss or radiation, remains challenging. Ideally, one would like to probe and vary QP dynamics in a highly coherent qubit, without requiring additional circuit elements or constraints that compromise its performance. Here we introduce such a technique, capable of measuring the QP dynamics of a qubit in operation and quantifying the processes of recombination, trapping, diffusion and background generation of QPs. With this technique, we directly measure the trapping of QPs by a single vortex, a basic property of superconductors. We demonstrate that QP trapping by vortices can suppress the background QP density, resulting in surprising net improvement of qubit coherence in spite of the well-known vortex flow dissipation [30] . In the following, we present time-domain measurements of QP relaxation in three-dimensional (3D) transmon qubits [31] over 2–3 orders of magnitude in density. We find that the QP dynamics can be dominated by either recombination or trapping effects depending on the device geometry and the resultant presence or absence of vortices. We demonstrate strong in-situ control of QP dynamics by magnetic field, and measure an intrinsic single-vortex trapping ‘power’ of (6.7±0.5) × 10 −2 cm 2 s −1 (that is, τ ss =1 s induced by a single vortex over an area of 6.7 × 10 −2 cm 2 ). Improvements of relaxation time ( T 1 ) and coherence time ( T 2E ) by more than a factor of 2 are observed in one geometric design of devices when the devices are cooled in a small magnetic field (10–200 mG). We measure a stray QP generation rate of about 1 × 10 −4 s −1 , suggesting the long coherence time of the widely adapted design of 3D transmons [12] , [31] , [32] , [33] may already be greatly assisted by unintentional vortices. Improved coherence by field-cooling, also being reported in superconducting planar resonators [34] and fluxonium qubits [35] during the preparation of our manuscript, can be definitively correlated with QP trapping rates of vortices as probed by our measurements of QP dynamics. Injection and measurement of QPs In our experiment, we inject QPs into two types of transmon qubits in a 3D cQED (circuit quantum electrodynamics) architecture [31] using only the existing microwave ports. Each transmon qubit comprises a single Al/AlO x /Al Josephson junction shunted by a large Al coplanar capacitor (electrodes) on a c -plane sapphire substrate. Type A devices are very similar to those in ref. 31 with a pair of large 500 × 250 μm 2 electrodes ( Fig. 1b ). The electrodes of type B devices are composed of a narrow (6–30 μm wide) coplanar gap capacitor and a pair of 80 × 80 μm 2 ‘pads’ (see Fig. 1c and Supplementary Fig. 1 ), but provide total capacitance and qubit Hamiltonian parameters very similar to type A devices. Chips containing one or two qubits are mounted in 3D aluminium or copper rectangular waveguide cavities ( Fig. 1a ) and all measurements are done in an Oxford cryogen-free dilution refrigerator at base temperature of 15–20 mK, with magnetic field shielding, infrared shielding and filtering described in ref. 32 . To inject QPs, similar to ref. 35 we apply a high-power microwave pulse at the bare cavity resonance frequency from the input port. The injection pulse creates about 10 5 circulating photons in the cavity, resulting in an oscillating voltage across the Josephson junction that exceeds the superconducting gap, and produces ~10 5 QPs per μs. The duration of the injection pulse is long enough (200–500 μs) so that the injected QPs can fully diffuse within the device, whereas the production and loss of QPs reach a dynamic balance. (See Supplementary Notes 1 and 2 for analysis of QP injection and diffusion.) 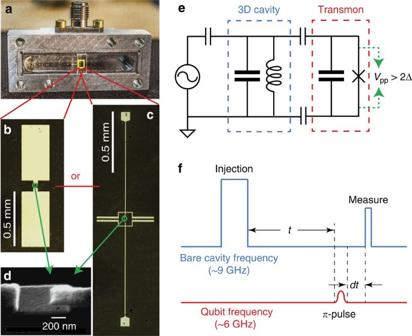Figure 1: Device and measurement schematics. (a) Photograph of half of a 3D aluminium cavity loaded with a transmon qubit. (b,c) Optical images of a type A device and a type B device. (d) Scanning electron microscope image of a Josephson junction located in between the two electrodes of a transmon. (e) Effective circuit of the cavity-qubit system. Injection of quasiparticles is achieved by applying a resonant microwave voltage to the 3D cavity capacitively coupled to the junction. (f) Pulse sequences for measuring the decay of quasiparticles based on qubitT1. A π-pulse is applied to excite the qubit from |g› to |e› at a variable delaytafter the injection pulse, followed by a readout pulse after another variable delay. Figure 1: Device and measurement schematics. ( a ) Photograph of half of a 3D aluminium cavity loaded with a transmon qubit. ( b , c ) Optical images of a type A device and a type B device. ( d ) Scanning electron microscope image of a Josephson junction located in between the two electrodes of a transmon. ( e ) Effective circuit of the cavity-qubit system. Injection of quasiparticles is achieved by applying a resonant microwave voltage to the 3D cavity capacitively coupled to the junction. ( f ) Pulse sequences for measuring the decay of quasiparticles based on qubit T 1 . A π-pulse is applied to excite the qubit from | g › to | e › at a variable delay t after the injection pulse, followed by a readout pulse after another variable delay . Full size image We use the recovery of the energy relaxation time ( T 1 ) of the qubit as a direct and calibrated probe of the decay of QP density. Standard microwave pulse sequences are applied to determine the qubit T 1 following a variable delay t after the QP injection ( Fig. 1f and Supplementary Note 3 ), from which we extract the qubit relaxation rate Γ=1/ T 1 as a function of t as shown in Fig. 2 . Despite possible heating due to the injection pulse, we find the effective temperature of the qubit and QP bath does not exceed 70 mK for the entire range of our measurement ( Supplementary Note 4 ), therefore thermal generation of QPs and spontaneous | g ›→| e › transition of the qubit can be neglected. We use x qp to represent the QP density near the Josephson junction normalized by the Cooper-pair density ( n cp ≈4 × 10 6 μm −3 for aluminium). It is related to the measured qubit decay rate by Γ( t )= Cx qp ( t )+Γ ex , where Γ ex is a constant qubit decay rate because of non-QP dissipation mechanisms, and is a calculated [6] and confirmed [31] constant involving only the superconducting gap Δ(≈180 μ e V) and the angular frequency of the transmon ω q (≈2 π ·6 GHz). As Γ ex is strictly bounded by the qubit relaxation rate without QP injection, Γ ex ≤Γ 0 =Γ( t →∞), for a significant range of the data, QP density can be approximated by x qp ( t )≈Γ( t )/ C . 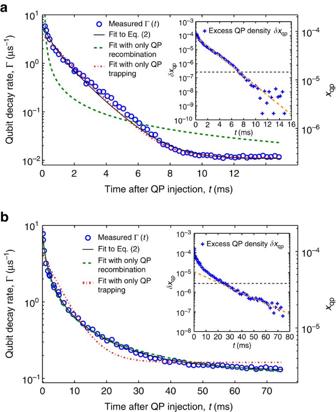Figure 2: Quasiparticle (QP) decay dynamics characterized by the recovery functional forms of qubit decay rate. Qubit energy decay rate Γ as a function of timetafter QP injection pulses and fits to various functional forms for Device A1 (a, dominated by trapping) and Device B1 (b, dominated by recombination) in separate aluminium 3D cavities. For illustration purposes, we labelxqp=Γ/Con the right axes, neglecting qubit relaxation from non-QP mechanisms that have a stringent bound Γex≤Γ0. Insets, replots of the Γ(t) data in main panels in the form of excess QP densityδxqpafter subtracting a background (whose magnitude Γ0/Cis shown by the black dashed line and is an upper bound ofx0). The magenta dashed line is guide to the eye of the exponential decay ofδxqpapproaching the steady state. Figure 2: Quasiparticle (QP) decay dynamics characterized by the recovery functional forms of qubit decay rate. Qubit energy decay rate Γ as a function of time t after QP injection pulses and fits to various functional forms for Device A1 ( a , dominated by trapping) and Device B1 ( b , dominated by recombination) in separate aluminium 3D cavities. For illustration purposes, we label x qp =Γ/ C on the right axes, neglecting qubit relaxation from non-QP mechanisms that have a stringent bound Γ ex ≤Γ 0 . Insets, replots of the Γ( t ) data in main panels in the form of excess QP density δx qp after subtracting a background (whose magnitude Γ 0 / C is shown by the black dashed line and is an upper bound of x 0 ). The magenta dashed line is guide to the eye of the exponential decay of δx qp approaching the steady state. Full size image Distinguishing between QP recombination and trapping The dynamics of the QP density x qp near the junction in the presence of recombination and trapping can be modelled by the following equation (see Supplementary Note 5 for details): The quadratic term describes the canonical QP recombination in pairs with a recombination constant r . The linear term describes trapping effects that localize or remove single QPs from tunnelling across the Josephson junction and inducing qubit relaxation. The effective trapping rate s depends not only on the property and density of the trapping sites, but also their geometric distribution and associated diffusion timescale. The constant term g describes QP generation rate by pair-breaking stray radiation or other unidentified sources [36] . If trapping is dominant ( s >> rx qp for most of the measured range of x qp ), then decay of x qp follows an exponential function. This is a surprisingly good approximation for the Γ( t ) we measured in Device A1 (of type A; red fit in Fig. 2a ). On the other hand, if recombination dominates, the decay of x qp follows a hyperbolic cotangent function, with initially a steep 1/ t decay crossing over to an exponential tail. We measure Γ( t ) in Device B1 (of type B) strikingly close to this limit (green fit in Fig. 2b ). To analyse both recombination and trapping more quantitatively, we solve equation (1) analytically, yielding a four parameter fit for Γ( t ) (black curves in Fig. 2 ): where x i is the initial injected QP density, Γ 0 = Cx 0 +Γ ex is the qubit relaxation rate without QP injection, consisting of contributions from both background QP density x 0 and other mechanisms. r ′ is a dimensionless fit parameter (0< r ′<1). Note that as t →∞, equation (2) approaches an exponential decay with time constant τ ss . The recombination constant r and the trapping rate s can be determined from these fit parameters ( Supplementary Note 5 ). For B1, a fit to equation (2) gives an exponential tail with τ ss =18±2 ms, a recombination constant r =1/(170±20 ns) and a weak trapping rate . For A1, we find s ≈1/ τ ss =1/(1.5±0.1 ms) and r =1/(105±30 ns), with the trapping term dominating most of the measurement range ( x qp <10 −4 ). The qualitative difference between the functional forms of QP decay in the two devices can be better illustrated by plotting the excess QP density because of QP injection, δx qp = x qp ( t )− x 0 , as a function of time ( Fig. 2 insets). For A1, the instantaneous QP decay rate indicated by the slope of δx qp ( t ) remains equal to its steady-state value (1/ τ ss ) even when the QP density is orders of magnitude higher than its background density (that is, when δx qp ( t )>>Γ 0 / C ≥ x 0 ). For B1, the slope increases significantly when δx qp ( t )> x 0 . Controlling QP dynamics by cooling in magnetic field Why do the two devices with identical material properties and similar qubit properties differ so much in QP relaxation dynamics? We attribute this to the trapping effect from vortices (regions with diminished superconducting gap) in the large electrodes in Device A1 despite the low level of residual field (B~1–2mG) achieved in our experiment by magnetic shielding. On the other hand, Device B1 is likely free of vortices because of the much narrower geometry of the electrodes. To test this hypothesis, we repeat Γ( t ) measurements in B1 after cooling the device through the critical temperature ( T c ) in a perpendicular magnetic field of variable magnitude B in either polarity. Indeed, as B increases, we observe significant acceleration of QP decay with increasingly pronounced single-exponential characteristics, indicating enhanced QP trapping ( Fig. 3a ). In comparison, changing the applied magnetic field at 20 mK does not produce measurable changes in QP dynamics. 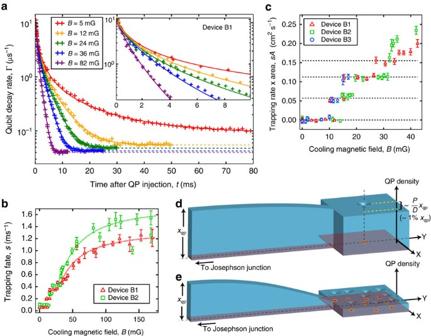Figure 3: Quasiparticle (QP) trapping by vortices. (a) Qubit decay rate Γ as a function of timetafter QP injection pulses for Device B1 cooled in a few selected magnetic fieldsB. Solid lines fit to equation (2). Dashed lines, background qubit decay rate indicating the ‘steady-state’T1of the qubit. Inset, zoom-in of the initial part of the decay. (b) QP trapping ratesas a function of cooling magnetic fieldBfor Devices B1 and B2. Each point represents data acquired after one field-cool thermal cycle (from above theTcof aluminium), with the error bars showing the 1 s.d. of fluctuations for repetitive measurements within each thermal cycle. Dotted lines, fits to the QP trapping/diffusion model. (c) QP trapping rate after subtracting a zero-vortex background and multiplying by the total area of the device, as a function ofBfor Devices B1, B2 and B3. Dashed lines are guides to the eye showing the discrete steps associated with 0, 1, 2 and 3 vortices. (d) Cartoon schematic (not to scale) of the near-homogeneous spatial distribution of QP density, represented by height of the blue volume (‘tank water level’), from the narrow wire (left) to the trapping pad (right) in a type B device when only one vortex is present. QP density near the vortex displays a small ripple with a relative depth on the order ofP/D≈1%. (e) Cartoon schematic (not to scale) of the QP density distribution with large number of vortices in the pad. The density at the trapping pad is much lower thanxqpnear the junction. Figure 3: Quasiparticle (QP) trapping by vortices. ( a ) Qubit decay rate Γ as a function of time t after QP injection pulses for Device B1 cooled in a few selected magnetic fields B . Solid lines fit to equation (2). Dashed lines, background qubit decay rate indicating the ‘steady-state’ T 1 of the qubit. Inset, zoom-in of the initial part of the decay. ( b ) QP trapping rate s as a function of cooling magnetic field B for Devices B1 and B2. Each point represents data acquired after one field-cool thermal cycle (from above the T c of aluminium), with the error bars showing the 1 s.d. of fluctuations for repetitive measurements within each thermal cycle. Dotted lines, fits to the QP trapping/diffusion model. ( c ) QP trapping rate after subtracting a zero-vortex background and multiplying by the total area of the device, as a function of B for Devices B1, B2 and B3. Dashed lines are guides to the eye showing the discrete steps associated with 0, 1, 2 and 3 vortices. ( d ) Cartoon schematic (not to scale) of the near-homogeneous spatial distribution of QP density, represented by height of the blue volume (‘tank water level’), from the narrow wire (left) to the trapping pad (right) in a type B device when only one vortex is present. QP density near the vortex displays a small ripple with a relative depth on the order of P / D ≈1%. ( e ) Cartoon schematic (not to scale) of the QP density distribution with large number of vortices in the pad. The density at the trapping pad is much lower than x qp near the junction. Full size image By fitting Γ( t ) to equation (2) at each cooling field, we find that: (i) the recombination constant r remains unchanged within fitting uncertainty, (ii) the trapping rate s increases in discrete and near-equal steps for small magnetic fields ( B ≲ 40 mG; Fig. 3c ), (iii) over a broader field range, s increases approximately linearly with B and saturates at ≳ 1 ms −1 at high field ( B ≳ 100 mG; Fig. 3b ). Our observed critical field threshold, B k , where the trapping rate s starts to increase, corresponds to the expected entry of the first vortex in one of the 80 × 80 μm 2 pads. B k can be estimated based on a thermodynamic analysis of a vortex in a thin superconducting disk [37] together with consideration of vortex creation-annihilation kinetics [38] , giving B k ~8 mG, close to our observed values of 11 mG for B1 in an Al cavity, 14 and 10 mG for other two devices of type B, B2 and B3, in Cu cavities. In comparison, B k for Device A1 is estimated to be about 0.5 mG, lower than the estimated residual field (and its possible inhomogeneity) of our setup and therefore cannot be observed experimentally. QP trapping by individual vortices The discrete trapping rates at small magnetic field are strongly suggestive of a fixed QP ‘trapping power’ for each individual vortex. We define trapping power, P , by modelling a vortex as a point object at a 2D spatial coordinate R 0 with a delta-function local trapping rate Pδ ( R − R 0 ). P could be more microscopically modelled as the product of QP trapping rate in the vortex core and an effective trapping area [28] , [34] ( Supplementary Note 6 ). However, the ‘trapping power’ representation offers the advantage of a general formulation without invoking any microscopic models. In the limit that diffusion is much faster than trapping, the total microscopic trapping power of N vortices, NP , manifests itself macroscopically as the product of the measured trapping rate and the total area, A , of the device, that is, sA = NP . For a small number of vortices, we observe quantized changes of sA products in steps of ~0.06 cm 2 s −1 consistent between all three systematically measured type B devices with up to 50% difference in device areas ( Fig. 3c ). In Fig. 3c , we have subtracted a relatively small (zero-vortex) background trapping rate that varies from device to device (zero field s <0.05 ms −1 for B1 but ~0.18 ms −1 for B3), whose origin remains to be explored in future studies. Assuming each step corresponds to the entry of one vortex (which is stochastically most probable and also suggested by the widths of the steps), and adjusting for the finite speed of QP diffusion ( Supplementary Note 5 ), we determine trapping power P =(6.7±0.5) × 10 −2 cm 2 s −1 as an intrinsic property of each individual vortex in our superconducting film. The reduced step heights and the eventual saturation of s at higher magnetic field can be fully explained by QP diffusion using realistic geometric parameters of our device ( Supplementary Note 5 ). When there are a large number of vortices in the pads, the apparent trapping rate s is limited by the diffusion time for QPs to reach the trapping pad from other regions of the device ( Fig. 3e ). The saturated trapping rate is higher for B2 because of the smaller volume of its gap capacitor. By fitting s as a function of B over a large range ( Fig. 3b ) for both devices, we determine the diffusion constant D =18±2 cm 2 s −1 for our Al film at 20 mK, consistent with the values measured in X-ray single-photon spectrometers adjusted for different temperature [25] . QP recombination constant Across seven devices ( Supplementary Table 1 ), we measure recombination constants r in the range of 1/(170 ns) to 1/(80 ns), consistent with the theoretical electron–phonon coupling time of aluminium τ 0 =438 ns (ref. 22 ) adjusting for the phonon-trapping effect [39] . Recombination-generated phonons can re-break Cooper pairs before escaping into the substrate, reducing the effective recombination constant by a factor F , giving . For our 80-nm bi-layer Al film on sapphire, the best estimate of F is in the range of 5–10 considering the strong acoustic mismatch at the interface [40] . The reported values of r for Al in the literature range from 1/(120 ns) to 1/(8 ns) [14] , [18] , [19] , [28] , [41] . The recombination constant we measured directly from the power-law decay characteristics is near the low end. It is comparable to r =1/(120 ns) extracted from DC steady-state injection measurements in extended Al films with similar thickness on sapphire [14] . Our measured value of r suggests the effect of recombination is extremely weak for the sparse QP background in typical superconducting qubits (recombination-resulted τ ss ~50 ms for x qp ~10 −6 ). Even one single vortex (occupying less than one-millionth of the total area of a type B device) can eliminate QPs much faster than the intrinsic recombination process, as demonstrated by the drastically different QP decay curves for 0 (red), 1 (orange) and 2 (green) vortices in Fig. 3a . Improved qubit coherence by vortices In strong correlation with the reduced QP lifetime because of vortex trapping, we observe dramatic improvement of qubit coherence as a result of the suppressed background QP density. Improved qubit T 1 is already demonstrated by the lower background Γ 0 in Fig. 3a at higher cooling field. This ‘steady-state’ T 1 of the qubit can also be measured separately without QP injection, which more than doubled from its zero-field value over a wide range of cooling magnetic field for both Devices B1 ( Fig. 4a ) and B2 ( Fig. 4b ). The coherence time with Hahn echo, T 2E , shows similar relative improvement because it is close to the limit of 2 T 1 . 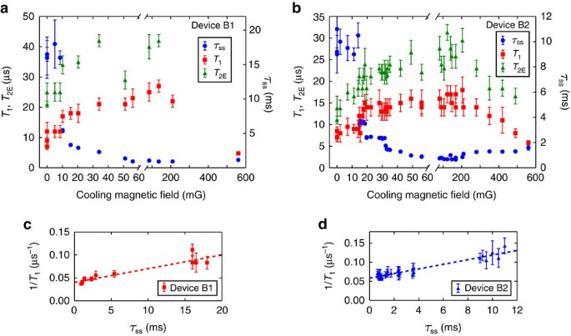Figure 4: Improved qubit coherence by cooling in magnetic field and its correlation with reduced quasiparticle (QP) lifetime. (a,b) Qubit steady-state relaxation timeT1, coherence time with echoT2Eand QP lifetimeτssas a function of cooling magnetic fieldBfor Devices B1 (a) and B2 (b). Each point represents data acquired after one field-cool thermal cycle, with the error bars showing the 1 s.d. of fluctuations for repetitive measurements within each thermal cycle. Note the discontinuous scale of thexaxes. (c,d) 1/T1versusτssas varied by cooling in different magnetic fields for B1 (c) and B2 (d). The dashed lines are linear fits based on equation (3), giving Γex=1/(26 μs),g=0.7 × 10−4s−1for B1 and Γex=1/(17 μs),g=1.3 × 10−4s−1for B2, respectively. Figure 4: Improved qubit coherence by cooling in magnetic field and its correlation with reduced quasiparticle (QP) lifetime. ( a , b ) Qubit steady-state relaxation time T 1 , coherence time with echo T 2E and QP lifetime τ ss as a function of cooling magnetic field B for Devices B1 ( a ) and B2 ( b ). Each point represents data acquired after one field-cool thermal cycle, with the error bars showing the 1 s.d. of fluctuations for repetitive measurements within each thermal cycle. Note the discontinuous scale of the x axes. ( c , d ) 1/ T 1 versus τ ss as varied by cooling in different magnetic fields for B1 ( c ) and B2 ( d ). The dashed lines are linear fits based on equation (3), giving Γ ex =1/(26 μs), g =0.7 × 10 −4 s −1 for B1 and Γ ex =1/(17 μs), g =1.3 × 10 −4 s −1 for B2, respectively. Full size image We can separate qubit loss mechanisms based on the linear relation between 1/ T 1 and τ ss (noting x 0 ≈ gτ ss ), where the intercept equals the qubit relaxation rate because of other loss mechanisms, and the slope reveals the stray QP generation rate g ( Fig. 4c,d ). In both B1 and B2, Γ ex is likely dominated by dielectric loss at the Al/Al 2 O 3 interface under the gap capacitor [42] . We find QP generation rate g ≈0.7–1.3 × 10 −4 s −1 in the two devices over several thermal cycles, or 0.3–0.6 QPs created per ms for every μm 3 of volume. Vortex flow dissipation The eventual decrease of T 1 and T 2E at high-magnetic field ( B ≳ 200 mG) can be attributed to vortices entering the gap capacitors where current density is high. Such dissipation due to vortex flow resistance has been well-known to degrade the quality factor of superconducting resonators and qubits [43] , [44] . Therefore, precautions such as multilayer magnetic shielding, specialized non-magnetic hardware and honeycomb-style device designs have been widely employed in the community to avoid vortices. However, here we have shown that the benefit of vortices in suppressing non-equilibrium QPs is not only relevant to practical devices, but can also significantly outweigh its negative impact if the locations of the vortices are optimized. In device A1 (or most type A devices, see Supplementary Table 1 ), our measured τ ss at nominally zero field implies the presence of about 20 vortices based on our measured single-vortex trapping power, consistent with its geometry assuming a residue magnetic field of 1–2 mG. Introducing more vortices to type A devices by cooling in an applied magnetic field can further reduce τ ss , but no clear improvement of qubit T 1 is observed. We attribute it to the limited range that τ ss can be varied (from its already small value at nominally zero field) and the vortex flow dissipation, which clearly reduces T 1 at B ≳ 30 mG ( Supplementary Note 7 ). Assuming both types of devices have similar g as they are shielded and measured in the same setup, it is plausible to infer that the long coherence times of the widely adopted type A 3D transmons would have been limited to much lower values without the assistance from QP trapping by unintentional vortices. In our work, for the first time, the interaction between QPs and a single vortex is measured. The single-vortex trapping power ( P ) is an intrinsic property of an aluminium film, and has the same dimension as the diffusion constant ( D ). The fact that we measure P / D ≈10 −2 implies that a QP can diffuse through a vortex with only a small (~1%) probability to be trapped. Despite a vortex being a topological defect with Δ=0 at its core, the spatial distribution of QP density is barely perturbed by the presence of a vortex, just like a small ‘ripple’ on the order of 1% deep in a flat ‘sea’ ( Fig. 3d , see Supplementary Note 8 for calculation). For a uniform film extended in 2D space, this relatively homogeneous QP distribution holds for all practical length scales at any density of vortices, so the trapping rate s can be simply computed from the total trapping power. In the high-magnetic field limit, this leads to s ∝ B with a linear coefficient P / φ 0 =0.3 μs −1 G −1 based on our measured P , close to the fitted value of 0.5 μs −1 G −1 in ref. 28 . Understanding and controlling the steady-state QP lifetime ( τ ss ) may be important for a variety of superconducting devices. For superconducting qubits and resonators, achieving short τ ss (either with vortices or potentially more efficient methods such as band-gap engineering or normal metal traps) to suppress the background QP density is desirable. In other devices such as kinetic inductance detectors [9] , [10] , it may be desirable to obtain a long QP lifetime. Our measured τ ss of 18 ms in a type B device is so far the longest reported in aluminium. Previous experiments in aluminium films showed that the expected exponential increase of τ ss with lower temperature saturates below 200 mK (refs 14 , 15 , 18 ) to about 3 ms at most [10] . To shed light on the mechanisms limiting τ ss in this regime of extremely low QP density (without intentional QP traps), our technique allows quantitative separation between QP recombination and any residual trapping effects. Our quantification of the weak recombination of background QPs and the single-vortex trapping extends our understanding of QP dynamics into the 10’s of millisecond regime, and thus sets a more stringent bound on possible additional mechanisms in limiting the QP lifetimes. To distinguish between recombination and trapping of QPs, our analysis relies critically on large dynamic range in x qp to achieve sufficient contrast between the functional forms of QP decay. A measurement near a steady state would observe the exponential tail of the decay, giving τ ss =1/( s +2 rx 0 ) without distinguishing between the two mechanisms. Such analysis of linear response has been traditionally carried out in time-domain measurements after photon pulses [15] , [19] , [23] , [25] . Noise spectroscopy measurements [15] , [19] by design are also limited to measuring the single timescale of τ ss . The experiment of Lenander et al . [20] introduced the use of qubit T 1 to probe QP dynamics, but the achieved dynamic range was below a factor of 4. The dynamic range of 2–3 orders of magnitude in our experiment has been made possible by a long T 1 time in 3D transmons, the effectiveness of our microwave injection technique and the geometric simplicity of an isolated aluminium island to eliminate out-diffusion. A significant stray QP generation rate of about 1 × 10 −4 s −1 has been measured in our study. Owing to the large device volume and relatively long integration time, our measured g should be considered a spatial-temporal average of QP generation rate. Quite remarkably, it agrees within a factor of 3 with the average QP generation rate in a much smaller fluxonium qubit [35] with a much shorter τ ss where there is evidence for the discreteness of QP numbers and QP generation events. This magnitude of QP generation rate, together with the weakness of recombination at low QP density, strongly suggests QP trapping should be an important ingredient for suppressing non-equilibrium x qp in superconducting qubits and other devices to further improve performance. Our method of extracting g utilizing the sensitivity of type B devices to QP generation should facilitate future identification of the QP generation source. The injection and measurement technique introduced in this work can be readily applied to nearly all cQED implementations without any modification to device structure or measurement circuit, and can play a crucial role in the future development of quantum circuits as a powerful probe of QP dynamics. How to cite this article: Wang, C. et al . Measurement and control of quasiparticle dynamics in a superconducting qubit. Nat. Commun. 5:5836 doi: 10.1038/ncomms6836 (2014).